Tonic excitation or inhibition is set by GABAAconductance in hippocampal interneurons Inhibition is a physiological process that decreases the probability of a neuron generating an action potential. The two main mechanisms that have been proposed for inhibition are hyperpolarization and shunting. Shunting results from increased membrane conductance, and it reduces the neuron-firing probability. Here we show that ambient GABA, the main inhibitory neurotransmitter in the brain, can excite adult hippocampal interneurons. In these cells, the GABA A current reversal potential is depolarizing, making baseline tonic GABA A conductance excitatory. Increasing the tonic conductance enhances shunting-mediated inhibition, which eventually overpowers the excitation. Such a biphasic change in interneuron firing leads to corresponding changes in the GABA A -mediated synaptic signalling. The described phenomenon suggests that the excitatory or inhibitory actions of the current are set not only by the reversal potential, but also by the conductance. GABA is the main inhibitory neurotransmitter in the adult brain. Synaptically released GABA activates postsynaptic GABA A receptors, which trigger fast inhibitory postsynaptic currents (IPSCs). Ambient GABA produces persistent activation of extrasynaptic GABA A receptors, which are responsible for the tonic current [1] , [2] , [3] . The tonic current is mediated by heterogeneous and plastic GABA A receptors [4] , [5] and is expressed in a cell-type specific manner in various brain structures, such as the hippocampus [6] , thalamus [7] , neocortex [8] and striatum [9] . Cell type-specific expression of the tonic current indicates the importance of this phenomenon for neuronal network operation, especially when the extracellular GABA concentration changes. Indeed, changes in ambient GABA levels are reported in both physiological (for example, during exploratory behaviour) and pathological (for example, epilepsy, pain) conditions [10] , [11] , [12] . The effect of GABA on cell excitability is largely determined by the reversal potential for Cl − , which is the major ion responsible for the GABA A current. In adult neurons, the intracellular Cl − concentration is kept low by developmentally regulated cotransporters [13] , [14] and sets a reversal potential for GABA A currents ( E GABA ) close to the resting membrane potential (RMP). The RMP and E GABA vary among cell types and even cell compartments [15] , [16] ; therefore, the effect of GABA can be either hyperpolarizing or depolarizing. Whereas hyperpolarization is the primary synaptic action of GABA on cortical principal neurons [17] , depolarizing effects of GABA are observed in interneurons in numerous circuits, including the hippocampus [18] , [19] , [20] , [21] , cerebellum [22] , and basolateral amygdala [23] ; as well as in striatal neurons [9] , [24] and peripheral nervous system neurons [25] . Because this depolarization is set by a small driving force for Cl − , the predominant effect of GABA A activation is thought to be shunting inhibition. Shunting inhibition is a conductance-dependent phenomenon and may not provide strong inhibitory effects on the cell at low GABA A conductances. In contrast, even a small depolarization of the neuronal membrane can trigger activation of some voltage dependent channels. In turn, activation of these channels can potentially bring the RMP to the action potential threshold. This raises the possibility that low depolarizing GABA A conductance can be excitatory whereas high conductance is inhibitory though shunting [26] . Previous reports suggested that voltage-dependent oscillations of the membrane potential in hippocampal interneurons could reach the action potential threshold and trigger cell firing [27] , [28] , [29] . Indeed, hippocampal CA1 stratum ( str. ) radiatum interneurons could fire spontaneous action potentials even when excitatory neurotransmission was blocked. Here we found that the firing frequency of these cells is bidirectionally regulated by ambient GABA concentrations. Low GABA concentrations increased both membrane potential fluctuations and cell firing; high concentrations decreased these two parameters below the control values. Biphasic effect of tonic conductance on interneuron firing We investigated the effect of tonic GABA A conductance on CA1 str. radiatum interneurons in mouse hippocampal slices and blocked ionotropic glutamate and GABA B receptors. Consistent with previous reports, gramicidin-perforated patch recordings showed that these cells have depolarizing E GABA (RMP, −71.4±2.7 mV n =5; E GABA , −62.4±2.7, n =5, P =0.003 paired t -test; Fig. 1a,b ) [18] , [19] , [20] , [21] . As expected, exogenous GABA produced a concentration-dependent increase in the tonic GABA A conductance (Δ g GABA , 0.41±0.08 nS, 0.72±0.09 nS, and 1.55±0.34 nS for 1, 5, and 50 μM GABA, respectively, n =8; Fig. 1c,d ) [3] , [6] . In cell-attached recordings, the interneurons could fire spontaneous action potentials despite the blockade of ionotropic glutamate receptors ( Supplementary Fig. S1 ). In contrast to the commonly held notion that GABA mediates inhibitory tonic conductance [1] , [2] , [30] , however, 1 μM GABA increased interneuron firing by 1.68±0.18 Hz ( n =7, P =0.028 paired t -test). Cell firing did not significantly change with 5 μM GABA (increase by 0.6±0.6 Hz, n =5, P =0.2 paired t -test), and significantly decreased with 50 μM GABA by 3.9±1.3 Hz ( n =5, P =0.023 paired t -test; Fig. 1e,f ). These findings suggest a biphasic effect of tonic GABA A conductance on cell excitability. Therefore, we established the inhibitory threshold conductance at which GABA switches its action from excitatory to inhibitory and the peak excitation conductance at which GABA produces maximal excitatory effect. We plotted the cell firing rate versus the corresponding tonic GABA A conductance ( g GABA =baseline tonic conductance+Δ g GABA ). The inhibitory threshold conductance (1.73 nS) and the peak excitation conductance (1.16 nS) were obtained from a second-order polynomial fit ( Fig. 1g ). These two parameters characterize the cell response to the change in ambient GABA concentration and are potentially important for computation within individual interneurons and local networks. 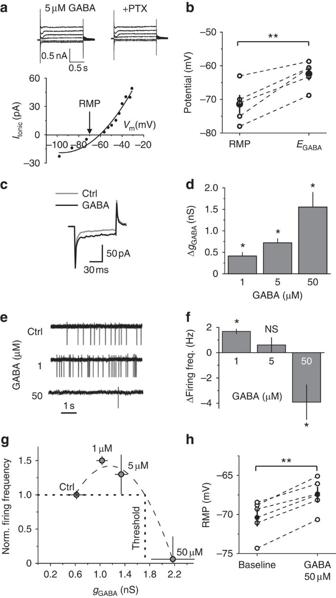Figure 1: The effect of ambient GABA on interneuron membrane properties and firing. (a) Top, Gramicidin-perforated patch recordings at voltage steps from −90 to −20 mV in 5 μM GABA and, thereafter 100 μM picrotoxin (+PTX) was added. Tonic GABAAcurrents at different voltages were calculated by subtracting the '+PTX'-currents from corresponding '5 μM GABA'-currents. Bottom: Tonic current (Itonic) versus membrane potential (Vm). Points were fitted with a second-order polynomial function to determineEGABA. Arrow marks RMP. (b) Summary data of RMP andEGABAshowing data from individual cells (n=5, empty circles) and mean values (black circles). (c) Five averaged current traces induced by −5 mV voltage step in control (ctrl) and in 50 μM GABA, demonstrating change in membrane conductance. (d) Summary plot of the GABA-induced change in membrane conductance (ΔgGABA) (n=7 for 1 μM GABA,n=5 for 5 μM GABA,n=5 for 50 μM GABA). (e) Cell-attached recordings from interneurons in control and in 1 and 50 μM GABA. (f) Summary plot of the change in firing frequency induced by GABA. (g) Summary plot of normalized firing frequency versus tonic GABAAconductance (gGABA) with a second order polynomial fit (dashed line). Dotted lines indicate the threshold conductance. (h) Effect of 50 μM GABA on RMP in individual cells (n=5, empty circles) and mean values (black circles). Error bars, s.e.m., **P<0.005, *P<0.05, NSP>0.05, pairedt-test. Figure 1: The effect of ambient GABA on interneuron membrane properties and firing. ( a ) Top, Gramicidin-perforated patch recordings at voltage steps from −90 to −20 mV in 5 μM GABA and, thereafter 100 μM picrotoxin (+PTX) was added. Tonic GABA A currents at different voltages were calculated by subtracting the '+PTX'-currents from corresponding '5 μM GABA'-currents. Bottom: Tonic current ( I tonic ) versus membrane potential ( V m ). Points were fitted with a second-order polynomial function to determine E GABA . Arrow marks RMP. ( b ) Summary data of RMP and E GABA showing data from individual cells ( n =5, empty circles) and mean values (black circles). ( c ) Five averaged current traces induced by −5 mV voltage step in control (ctrl) and in 50 μM GABA, demonstrating change in membrane conductance. ( d ) Summary plot of the GABA-induced change in membrane conductance (Δ g GABA ) ( n =7 for 1 μM GABA, n =5 for 5 μM GABA, n =5 for 50 μM GABA). ( e ) Cell-attached recordings from interneurons in control and in 1 and 50 μM GABA. ( f ) Summary plot of the change in firing frequency induced by GABA. ( g ) Summary plot of normalized firing frequency versus tonic GABA A conductance ( g GABA ) with a second order polynomial fit (dashed line). Dotted lines indicate the threshold conductance. ( h ) Effect of 50 μM GABA on RMP in individual cells ( n =5, empty circles) and mean values (black circles). Error bars, s.e.m., ** P <0.005, * P <0.05, NS P >0.05, paired t -test. Full size image According to the above definition of the peak excitation conductance an increase in the tonic GABA A conductance further from this point should decrease the cell firing rate and vice versa. Indeed, a low dose of the GABA A antagonist picrotoxin (1 μM) reversed the inhibitory effect of 10 μM GABA by partial reduction of the tonic GABA A conductance, presumably setting it closer to the peak excitation ( Supplementary Fig. S2 ). It should be noted that picrotoxin at this concentration has only a minor effect on IPSCs [6] . This finding is consistent with our previous report demonstrating an increase in hippocampal interneuron firing in guinea pigs by partially reducing the tonic conductance [6] . Baseline tonic GABA A conductance in guinea pig interneurons is almost twice that in mice (guinea pigs, 1.1±0.3 nS, n =7 versus mice, 0.62±0.16 nS, n =7) [6] and could be above the excitation peak conductance in these animals, even if still below the inhibitory threshold conductance (excitatory GABA action). The inactivation of Na + channels is an alternative explanation for the biphasic effect of tonic GABA A depolarization. This explanation for the inhibitory effect of depolarizing GABA was previously suggested for neurons in the peripheral nervous system [31] . In fact, GABA could not provide strong depolarization to hippocampal interneurons, even at high conductances ( E GABA ~10 mV above RMP). 50 μM GABA produced only 3.1±0.1 mV ( n =5, P =0.001 paired t -test) of depolarization in perforated-patch experiments ( Fig. 1h ). In whole-cell current clamp recordings, we tested the effect of a depolarizing block on the interneuron firing by injecting different amounts of constant current. At first, cell firing increased with the depolarization, but after the depolarization reached −38.7±4.1 mV (~26 mV above RMP, n =5), the firing rate began to decrease, presumably due to inactivation of Na + channels. This finding indicates that the small amount of depolarization produced by ambient GABA is unlikely to produce a significant depolarizing block in hippocampal interneurons. We cannot completely rule out this possibility, however, because the depolarizing effect of GABA can be larger in the axon initial segment, as it has been demonstrated in principle cells in the context of axo-axonic synaptic connections [16] , [32] . The small depolarization produced by tonic GABA A conductances raises the question that whether it is sufficient to reach the action potential threshold. Consistent with previous reports, the action potential threshold (the value of membrane potential when the first derivative of potential was 30 mV/ms) estimated in whole-cell current clamp recordings was −43.9±2.3 mV ( n =8) [27] . Indeed, the small depolarization produced by tonic GABA A conductance cannot reach this value. The action potential measurements, however, are commonly obtained in the cell soma although the action potential threshold can be lower in the axon trigger zone. Moreover, neuron firing can be triggered not by constant depolarization, but through the enhancement of voltage-dependent membrane potential fluctuations characteristic of interneurons [29] , [33] . Indeed, GABA produced a biphasic effect on the standard deviation (s.d.) of the RMP recorded in perforated-patch experiments: 1 μM GABA increased s.d. by 25±8% ( n =5, P =0.04 paired t -test), 5 μM produced an insignificant decrease of 10±10% ( n =7, P =0.19, paired t -test), and 50 μM decreased the s.d. by 24±9% ( n =6, P =0.03 paired t -test). The observed decrease in the RMP fluctuations produced by 50 μM GABA was consistent with the previously reported observations in cell attached recordings [21] . Thus, our results point that low tonic GABA A conductance depolarizes the cell and enhances voltage-dependent fluctuations of the RMP, which can trigger action potentials. When the conductance increases, however, it shunts the fluctuations and prevents cell firing. If this is the case, such a mechanism should work not only in hippocampal interneurons, but also in any neuron with depolarizing GABA. We addressed this issue by developing a simple computer simulation on a cylindrical model cell lacking any interneuron-specific features. The excitability of this cell was based on the Hodgkin–Huxley model with the kinetics of Na + and K + channels assuming stochastic opening and closing (Methods). The cell also contained stochastic A-type K + channels [34] . Under baseline conditions, the cell received no synaptic input and generated no action potentials, but did show small fluctuations in the RMP ( Fig. 2a ). A tonic GABA A conductance ( g GABA =0–0.2 mS cm -2 ) with depolarizing E GABA (10.2 mV above RMP) was then introduced. This produced a biphasic change in the cell firing frequency that was dependent on the g GABA amplitude, similar to the effect observed in hippocampal interneurons ( Fig. 2a,b ). The density of Na + channels was then reduced from 50 μm −2 (in initial model) to 25 μm −2 to prevent the model cell from spiking, which allowed us to observe the effect of g GABA on the RMP fluctuations ( Fig. 2c ). The RMP s.d. initially increased with cell depolarization, and then decreased regardless of the membrane potential ( Fig. 2d ). Interestingly, the biphasic changes in the cell firing frequency and in the RMP fluctuations were not due to the inactivation of Na + channels. The depolarizing current injections did not produce any biphasic effect on the above parameters at the same RMP range that was produced by g GABA ( Fig. 2e–h ). This model demonstrates that the described phenomenon does not require any specific cell anatomy, subcellular gradients of E GABA , or inactivation of Na + channels; and can be achieved with a limited number of voltage-dependent conductances. 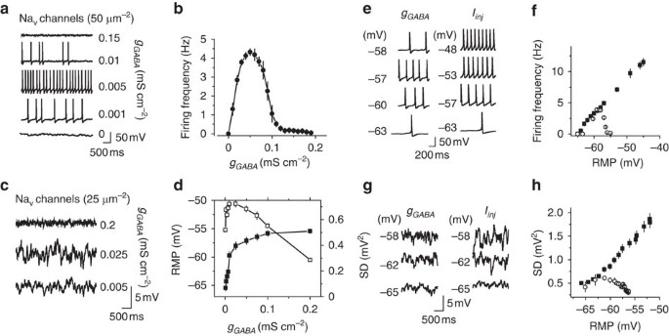Figure 2: The effect of depolarizing tonic GABAAconductance on a model neuron. (a) Sample traces of the cell firing induced bygGABA. (b) Summary plot of the cell firing frequency versusgGABA(n=10) (c) Sample traces of the effect ofgGABAon RMP fluctuations set by stochastic channel openings. The Na+channel density was reduced by half compared with panelato avoid cell firing. (d) Summary plot of RMP (black squares,n=10) and RMP standard deviation (s.d., white squares,n=10) versusgGABA. (e) Representative traces of membrane potential at different RMPs produced bygGABA(left panel) and byIinj(right panel). (f) Summary data of the change in the model cell firing at different RMPs set bygGABA(empty circles,n=10) and byIinj(black squares,n=10). (g) Representative traces of membrane potential at different RMPs produced bygGABA(left panel) and byIinj(right panel).gNawas reduced by half to prevent the cell from firing. (h) Mean standard deviation of RMP (s.d.) at different RMPs set bygGABA(empty circles,n=10) and byIinj(black squares,n=10). Error bars, s.e.m. Figure 2: The effect of depolarizing tonic GABA A conductance on a model neuron. ( a ) Sample traces of the cell firing induced by g GABA . ( b ) Summary plot of the cell firing frequency versus g GABA ( n =10) ( c ) Sample traces of the effect of g GABA on RMP fluctuations set by stochastic channel openings. The Na + channel density was reduced by half compared with panel a to avoid cell firing. ( d ) Summary plot of RMP (black squares, n =10) and RMP standard deviation (s.d., white squares, n =10) versus g GABA . ( e ) Representative traces of membrane potential at different RMPs produced by g GABA (left panel) and by I inj (right panel). ( f ) Summary data of the change in the model cell firing at different RMPs set by g GABA (empty circles, n =10) and by I inj (black squares, n =10). ( g ) Representative traces of membrane potential at different RMPs produced by g GABA (left panel) and by I inj (right panel). g Na was reduced by half to prevent the cell from firing. ( h ) Mean standard deviation of RMP (s.d.) at different RMPs set by g GABA (empty circles, n =10) and by I inj (black squares, n =10). Error bars, s.e.m. Full size image Synaptic GABA A currents are inhibitory Our findings suggest that whereas a low tonic GABA A conductance can be excitatory, synaptic signalling mediated by high GABA A conductance should provide shunting inhibition in hippocampal interneurons. To test this, we produced stimulations with an extracellular electrode placed proximally to the recorded cell in the str. radiatum . The recordings were performed in the presence of ionotropic glutamate and GABA B receptor antagonists. First, in whole-cell mode, we recorded the evoked GABA A -mediated postsynaptic current (PSC) induced in CA1 interneurons by 50-μA, 200-μs stimulus ( Supplementary Fig. S3 ). We then estimated the postsynaptic conductance (PSG) required to generate such a PSC according using the following formula: PSG=PSC/( E GABA − V hold ), where V hold is the holding potential (−70 mV). The PSG peak conductance 4.6±0.8 nS ( n =7, Fig. 3a ) was significantly larger than the conductance required to reach the inhibitory threshold conductance from the baseline tonic GABA A conductance (1.1 nS, calculated as the difference between the inhibitory threshold conductance and baseline tonic GABA A conductance, Fig. 1g ). Moreover, the synaptic conductance calculated from PSCs, recorded in the soma, was probably underestimated because some synaptic currents originate from the distal dendrites. Second, we recorded CA1 interneuron firing in the cell-attached mode and produced extracellular stimulation as described above. The time between the stimulus and preceding spike ( t ps ) was assumed to be random; the time between the stimulus and the succeeding spike ( t ss ) was influenced by the PSG. The mean t ps and t ss were compared for each cell ( Fig. 3b ). Consistent with the inhibitory synaptic effect, the t ss was almost twice as large as the t ps ( t ss / t ps , 1.96±0.55, n =6, P =0.011 paired t -test). The difference between t ps and t ss was completely blocked by 100 μM picrotoxin ( t ss − t ps , 126±14.7 ms in control and −7.8±35 ms in picrotoxin, n =5, P =0.02 paired t -test; Fig. 3c ). These data support the notion that GABA A -mediated PSGs in interneurons are inhibitory (IPSGs). Therefore, we use the term spontaneous inhibitory PSCs (sIPSCs) in the following sections for consistency. An alternative explanation for the inhibitory effect of synaptic GABA is that the site of action is different from that of tonic conductance. In a separate set of experiments, we tested the effect of a GABA puff (100 μM×100 ms). Similar to synaptic stimulation, the GABA puff increased the t ss by a factor of two ( t ss / t ps , 1.99±0.31, n =4, P =0.005 paired t -test; Fig. 3d ). Because puff application produces a local transient increase in GABA, which activates both synaptic and extrasynaptic GABA A receptors, this finding suggests that the conductance magnitude is more important than the site of action. 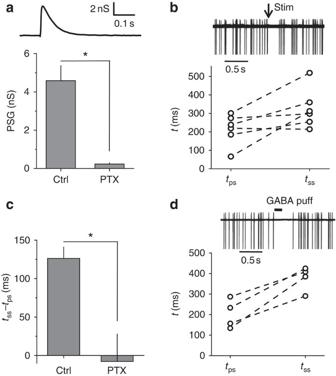Figure 3: Evoked GABAAPSG and 100 μM GABA puff are inhibitory. (a) Top: sample trace of calculated GABAAmediated PSG. Bottom, Summary plot of averaged peak PSG in control (ctrl) and in 100 μM picrotoxin (PTX) (n=7). (b) Top: Five superimposed cell-attached recordings with synaptic stimulation (arrow). Bottom: Plot of averaged preceding spike (tps) and succeeding spike (tss) intervals in 6 individual cells. (c) Difference betweentssandtpsin control (ctrl) and in 100 μM picrotoxin (PTX) (n=5). (d) Top: 5 superimposed cell-attached recordings with 100 μM GABA puff. Bottom: plot of averaged preceding spike (tps) and succeeding spike (tss) intervals in four individual cells. Error bars, s.e.m., *P<0.05, pairedt-test. Figure 3: Evoked GABA A PSG and 100 μM GABA puff are inhibitory. ( a ) Top: sample trace of calculated GABA A mediated PSG. Bottom, Summary plot of averaged peak PSG in control (ctrl) and in 100 μM picrotoxin (PTX) ( n =7). ( b ) Top: Five superimposed cell-attached recordings with synaptic stimulation (arrow). Bottom: Plot of averaged preceding spike ( t ps ) and succeeding spike ( t ss ) intervals in 6 individual cells. ( c ) Difference between t ss and t ps in control (ctrl) and in 100 μM picrotoxin (PTX) ( n =5). ( d ) Top: 5 superimposed cell-attached recordings with 100 μM GABA puff. Bottom: plot of averaged preceding spike ( t ps ) and succeeding spike ( t ss ) intervals in four individual cells. Error bars, s.e.m., * P <0.05, paired t -test. Full size image Biphasic changes in GABAergic synaptic signalling Tonic GABA A conductance is commonly referred as 'tonic inhibition' [1] , [2] , [30] and therefore its function in neuronal networks is thought to be unidirectional. Here we demonstrate that tonic GABA A conductance has a biphasic effect on the hippocampal interneuron firing rate. Interneurons are a diverse group of cells and each class of interneurons has a different function in the local network [35] . The amount of tonic GABA A conductance also varies among interneuron types [8] . Thus, our sample of interneurons does not characterize the tonic GABA A current in all classes of interneurons and cannot be used to predict the effect of ambient GABA on the CA1 network. Therefore, we recorded the sIPSC frequency directly in CA1 pyramidal neurons, which are the final targets of the CA1 interneurons and generate the major hippocampal output. Consistent with the biphasic change in interneuron firing, 1 μM GABA increased sIPSC frequency in the pyramidal cells by 1.5±0.5 Hz ( n =11, P =0.005 paired t -test), 5 μM GABA did not produce a significant change (increase by 0.25±0.55 Hz; n =9, P =0.34 paired t -test), and 50 μM GABA reduced the frequency by 1.2±0.4 Hz ( n =6, P =0.036 paired t -test; Fig. 4a,b ). In this set of experiments, we used relatively high concentrations of exogenous GABA (up to 50 μM). Although it is unlikely that all the GABA reached the neurons deep in the tissue because of its efficient uptake, it is still possible that some of the synaptic GABA A receptors were recruited or desensitised, and the activation of presynaptic GABA A receptors affected the probability of GABA release. To rule out these possibilities, we recorded action-potential independent miniature IPSCs (mIPSCs) under control conditions in the presence of 1 μM tetrodotoxin (Na + channel blocker) and then added 1, 5 or 50 μM GABA ( Supplementary Fig. S4 ). Neither the amplitude nor frequency of the mIPSCs changed significantly, suggesting the lack of synaptic GABA A receptor activation/desensitisation and the lack of an effect on GABA release probability, respectively. 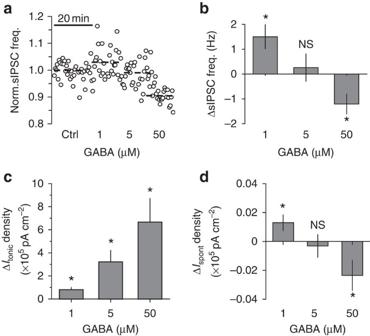Figure 4: Effect of ambient GABA on sIPSC and tonic current in CA1 pyramidal neurons. (a) Normalized sIPSC frequency in CA1 pyramidal neuron in control (ctrl) and after application of 1, 5 and 50 μM GABA. (b) Summary plot of the change in sIPSC frequency induced by GABA (n=11 for 1 μM GABA,n=9 for 5 μM GABA,n=6 for 50 μM GABA). (c) Summary plot of the change in tonic GABAAcurrent (ΔItonic) density recorded in 1, 5 and 50 μM GABA (n=10). (d) Summary plot of the change in time-averaged phasic current (ΔIspont) density recorded in 1, 5 and 50 μM GABA (n=10). Error bars, s.e.m., *P<0.05, NSP>0.05, pairedt-test. Figure 4: Effect of ambient GABA on sIPSC and tonic current in CA1 pyramidal neurons. ( a ) Normalized sIPSC frequency in CA1 pyramidal neuron in control (ctrl) and after application of 1, 5 and 50 μM GABA. ( b ) Summary plot of the change in sIPSC frequency induced by GABA ( n =11 for 1 μM GABA, n =9 for 5 μM GABA, n =6 for 50 μM GABA). ( c ) Summary plot of the change in tonic GABA A current (Δ I tonic ) density recorded in 1, 5 and 50 μM GABA ( n =10). ( d ) Summary plot of the change in time-averaged phasic current (Δ I spont ) density recorded in 1, 5 and 50 μM GABA ( n =10). Error bars, s.e.m., * P <0.05, NS P >0.05, paired t -test. Full size image Because of efficient GABA uptake, the tonic GABA A current is either absent in pyramidal cells or significantly smaller than that in interneurons [4] , [6] . Ambient GABA, however, can increase tonic GABA A current in these cells. Indeed, 1, 5 and 50 μM GABA produced a dose-dependent increase in the tonic GABA A current ( Fig. 4c ). This increase was two orders of magnitude larger than the change in the time-averaged current mediated by sIPSCs ( I spont ), which was calculated as mean charge transfer of sIPSCs multiplied by their frequency [6] ( Fig. 4d ). Thus, the overall effect of bath-applied GABA on the excitability of CA1 pyramidal neurons was dominated by tonic inhibition (Discussion). We next investigated the conditions under which ambient GABA is decreased. Reduced tonic conductance correlates with low firing rate We used a mouse lacking one of the two major GABA synthesizing enzymes, 65 kDa glutamic acid decarboxylase (GAD65−/−). This mouse develops an ambient GABA deficit in the brain after the first month of life [36] , [37] . Consistent with the reduced extracellular GABA, the tonic GABA A current density was two times smaller in CA1 str. radiatum interneurons of GAD65−/− mice than in wild-type (WT) mice interneurons (GAD65−/−, 1.5±0.3×10 5 pA cm −2 , n =7 versus WT, 3.2±0.6×10 5 pA cm −2 , n =10; P =0.037; Fig. 5a,b ). Surprisingly, we detected no difference in the magnitude of the tonic currents between the WT and GAD65−/− CA1 pyramidal neurons ( Fig. 5c,d ). It is possible that under baseline conditions, ambient GABA does not reach the receptors on these cells [6] and the small tonic current is mediated by agonist-independent spontaneous openings of GABA A receptors [38] , [39] . 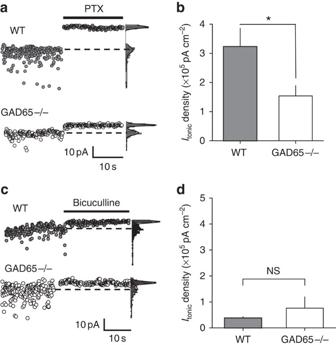Figure 5: Tonic GABAAcurrent in GAD65−/− interneurons and pyramidal cells. (a) Change inIholdin WT and GAD65−/− interneurons produced by 100 μM picrotoxin (PTX). Right panels: Current histograms with Gaussian fits of recorded current. Dashed lines indicate theIholdobtained from the peaks of the fits. (b) Summary plot of tonic GABAAcurrent (Itonic) density in interneurons (n=7 for GAD65−/−,n=10 for WT). (c) Change inIholdin WT and GAD65−/− pyramidal cells produced by 10 μM bicuculline. Right panels: same as ina. (d) Summary plot of tonic GABAAcurrent (Itonic) density in WT (n=6) and GAD65−/− (n=4) pyramidal cells. Error bars, s.e.m., NSP>0.05, *P<0.05, unpairedt-test. Figure 5: Tonic GABA A current in GAD65−/− interneurons and pyramidal cells. ( a ) Change in I hold in WT and GAD65−/− interneurons produced by 100 μM picrotoxin (PTX). Right panels: Current histograms with Gaussian fits of recorded current. Dashed lines indicate the I hold obtained from the peaks of the fits. ( b ) Summary plot of tonic GABA A current ( I tonic ) density in interneurons ( n =7 for GAD65−/−, n =10 for WT). ( c ) Change in I hold in WT and GAD65−/− pyramidal cells produced by 10 μM bicuculline. Right panels: same as in a . ( d ) Summary plot of tonic GABA A current ( I tonic ) density in WT ( n =6) and GAD65−/− ( n =4) pyramidal cells. Error bars, s.e.m., NS P >0.05, * P <0.05, unpaired t -test. Full size image GABA (5 μM) induced a similar rise in the holding current in GAD65−/− and WT interneurons, indicating that the smaller tonic current in knockout animals was not due to a change in their sensitivity to ambient GABA ( Fig. 6a,b ). Consistent with our previous report [6] , 100 nM zolpidem, a benzodiazepine site agonist, enhanced the tonic GABA A current and increased the sIPSC decay time in WT interneurons, suggesting that these currents were mediated by γ2-subunit-containing GABA A receptors ( Fig. 6c–f ). Zolpidem had a similar effect in GAD65−/− interneurons, pointing to an unchanged pharmacological profile of GABA A receptors in these animals [40] . Also consistent with a previous report [41] , the amplitude, kinetics and frequency of mIPSCs was not significantly different in GAD65−/− interneurons compared with WT interneurons ( Supplementary Fig. S5 ), suggesting that synaptic signalling was intact under resting conditions. This finding does not exclude, however, the possibility that synaptic GABA A signalling differs between the two genotypes during sustained synaptic activation induced by prolonged electrical stimulation, as previously reported [41] . Because we did not deliver prolonged stimulation to the slices, this phenomenon is unlikely to contribute to the difference in the tonic currents. 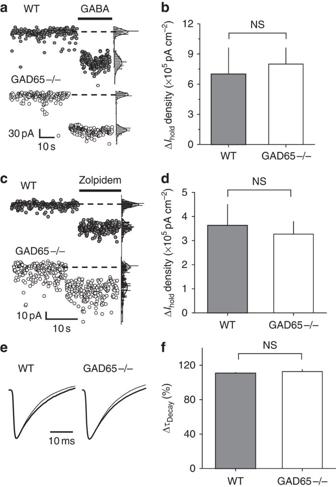Figure 6: WT and GAD65−/− interneurons equally respond to 5 μM GABA and 100 nM zolpidem. (a) Change inIholdin WT and GAD65−/− interneurons produced by 5 μM GABA. Right panels: current histograms with Gaussian fits of recorded current. Dashed lines indicate theIholdobtained from the peaks of the fits. (b) Summary plot of the change inIholddensity induced by 5 μM GABA in WT (n=10) and GAD65−/− (n=5) interneurons. (c) Change inIholdin WT and GAD65−/− interneurons produced by 100 nM zolpidem. Right panels: same as ina. (d) Summary plot of the change inIholddensity induced by zolpidem in WT (n=7) and GAD65−/− (n=7) interneurons. (e) Mean peak scaled sIPSCs recorded from WT and GAD65−/− interneurons without (thin trace) or with 100 nM zolpidem (thick trace). (f) Summary plot of the change in the sIPSC decay time constant (decay) induced by zolpidem in WT (n=7) and GAD65−/− (n=7) interneurons. Error bars, s.e.m., NSP>0.05, unpairedt-test. Figure 6: WT and GAD65−/− interneurons equally respond to 5 μM GABA and 100 nM zolpidem. ( a ) Change in I hold in WT and GAD65−/− interneurons produced by 5 μM GABA. Right panels: current histograms with Gaussian fits of recorded current. Dashed lines indicate the I hold obtained from the peaks of the fits. ( b ) Summary plot of the change in I hold density induced by 5 μM GABA in WT ( n =10) and GAD65−/− ( n =5) interneurons. ( c ) Change in I hold in WT and GAD65−/− interneurons produced by 100 nM zolpidem. Right panels: same as in a . ( d ) Summary plot of the change in I hold density induced by zolpidem in WT ( n =7) and GAD65−/− ( n =7) interneurons. ( e ) Mean peak scaled sIPSCs recorded from WT and GAD65−/− interneurons without (thin trace) or with 100 nM zolpidem (thick trace). ( f ) Summary plot of the change in the sIPSC decay time constant ( decay ) induced by zolpidem in WT ( n =7) and GAD65−/− ( n =7) interneurons. Error bars, s.e.m., NS P >0.05, unpaired t -test. Full size image In contrast to GABA A receptor knockout animals [42] , we found no changes in the non-GABA-mediated holding current in GAD65−/− interneurons, which suggests a lack of compensatory changes in the resting membrane conductances ( Fig. 7a ). The RMP (−70.6±2.5 mV, n =5) and E GABA (−59.2±1.8 mV, n =5, P =0.039 compared with RMP, paired t -test) in GAD65−/− interneurons were not significantly different from the RMP and E GABA in WT cells. 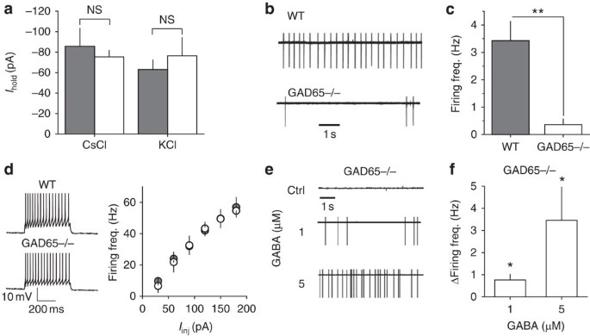Figure 7: Analysis of GAD65−/− interneurons. (a) Summary ofIholdrecorded in WT (shaded columns) and GAD65−/− (open columns) interneurons voltage-clamped at −60 mV loaded with CsCl (GAD65−/−n=8; WTn=13) and with KCl (GAD65−/−n=5; WTn=7) in the presence of 100 μM picrotoxin. (b) Cell-attached recordings from WT and GAD65−/− interneurons (without picrotoxin). (c) Summary plot of firing frequency in WT and GAD65−/− interneurons (n=7) obtained under the same conditions as forb. (d) Left panel: Action potentials recorded in response to depolarizing current steps (90 pA; 500 ms) in whole-cell current-clamp mode from WT and GAD65−/− interneurons in the presence of 100 μM picrotoxin. Right panel: Summary plot of action potential frequency recorded during depolarizing steps varying from 30 to 180 pA (input–output characteristics) in GAD65−/− (n=5) and WT (n=4) interneurons. (e) Cell-attached recordings from GAD65−/− interneuron in control (ctrl) and in 1 and 5 μM GABA (without picrotoxin). (f) Summary plot of the change in firing frequency induced by GABA in GAD65−/− interneurons obtained under the same conditions as fore. Error bars, s.e.m., **P<0.005, *P<0.05, NSP>0.05, unpaired (aandc) and paired (f)t-test. Figure 7: Analysis of GAD65−/− interneurons. ( a ) Summary of I hold recorded in WT (shaded columns) and GAD65−/− (open columns) interneurons voltage-clamped at −60 mV loaded with CsCl (GAD65−/− n =8; WT n =13) and with KCl (GAD65−/− n =5; WT n =7) in the presence of 100 μM picrotoxin. ( b ) Cell-attached recordings from WT and GAD65−/− interneurons (without picrotoxin). ( c ) Summary plot of firing frequency in WT and GAD65−/− interneurons ( n =7) obtained under the same conditions as for b . ( d ) Left panel: Action potentials recorded in response to depolarizing current steps (90 pA; 500 ms) in whole-cell current-clamp mode from WT and GAD65−/− interneurons in the presence of 100 μM picrotoxin. Right panel: Summary plot of action potential frequency recorded during depolarizing steps varying from 30 to 180 pA (input–output characteristics) in GAD65−/− ( n =5) and WT ( n =4) interneurons. ( e ) Cell-attached recordings from GAD65−/− interneuron in control (ctrl) and in 1 and 5 μM GABA (without picrotoxin). ( f ) Summary plot of the change in firing frequency induced by GABA in GAD65−/− interneurons obtained under the same conditions as for e . Error bars, s.e.m., ** P <0.005, * P <0.05, NS P >0.05, unpaired ( a and c ) and paired ( f ) t -test. Full size image Consistent with the excitatory effect of baseline tonic GABA A conductance, the firing frequency of GAD65−/− interneurons (0.023±0.01 Hz, n =7) was significantly lower than that of WT cells (3.2±0.7 Hz, n =7; P <0.001 compared with WT) ( Fig. 7b,c ). When GABA A receptors were blocked, the excitability of the GAD65−/− interneurons was not different from the WT cells, ruling out the possibility that compensatory changes were responsible for the reduced firing rate of these cells ( Fig. 7d ). If a reduced firing rate of GAD65−/− interneurons results from the decreased tonic GABA A conductance, exogenous GABA should rescue it. Indeed, bath application of 1 μM GABA increased the firing rate of GAD65−/− interneurons by 0.8±0.3 Hz ( n =6, P =0.015 paired t -test). In contrast to WT interneurons, 5 μM GABA further increased the firing rate of GAD65−/− interneurons by 3.5±1.5 Hz ( n =7, P =0.03 paired t -test; Fig. 7e,f ). This effect was due to lower baseline tonic conductance in GAD65−/− (0.31±0.12 nS, n =9) than that in WT (0.62±0.16 nS, n =7, P =0.042 for difference with GAD65−/−) interneurons. Both 1 and 5 μM GABA resulted in an increase in tonic conductance (Δ g GABA , 0.48±0.07 nS, n =9 and 1.07±0.15 nS, n =9, respectively) within the range of excitatory GABA action ( Fig. 1g ). This finding further supports the notion that the decreased firing rates of GAD65−/− interneurons are due to decreased tonic GABA A excitation. We then compared the baseline frequency of spontaneous action potential-dependent IPSCs (aIPSCs=sIPSCs—mIPSCs) in WT and GAD65−/− neurons to estimate the effect of an ambient GABA deficit on synaptic GABA A signalling driven by interneuron firing. Consistent with interneuron firing rates, the frequency of aIPSCs in WT pyramidal cells (1.2±0.4 Hz, n =4) was significantly higher than the frequency of the practically absent aIPSCs in GAD65−/− pyramidal cells (0.1±0.4 Hz, n =6, P =0.041 compared to WT; Fig. 8a ). A similar difference in the frequency of the aIPSCs was observed in the interneurons (WT, 1.1±0.3 Hz, n =13; GAD65−/−, −0.1±0.5 Hz, n =9, P =0.013; Fig. 8b ). 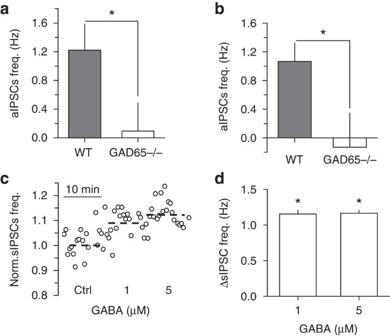Figure 8: GABAAmediated synaptic signalling in GAD65−/− CA1 neurons. (a,b) Summary plots of aIPSCs frequency in WT and GAD65−/− pyramidal cells (n=4 for WT,n=6 for GAD65−/−) and interneurons (n=13 for WT,n=9 for GAD65−/−), respectively. (c) Normalized sIPSC frequency in GAD65−/− pyramidal neuron in control (ctrl) and after 1 and 5 μM GABA application. (d) Summary plot of the change in sIPSC frequency by GABA in GAD65−/− pyramidal cells (n=8 for 1 μM GABA,n=6 for 5 μM GABA). Error bars, s.e.m., *P<0.05, unpaired (a,b) and paired (d)t-test. Figure 8: GABA A mediated synaptic signalling in GAD65−/− CA1 neurons. ( a , b ) Summary plots of aIPSCs frequency in WT and GAD65−/− pyramidal cells ( n =4 for WT, n =6 for GAD65−/−) and interneurons ( n =13 for WT, n =9 for GAD65−/−), respectively. ( c ) Normalized sIPSC frequency in GAD65−/− pyramidal neuron in control (ctrl) and after 1 and 5 μM GABA application. ( d ) Summary plot of the change in sIPSC frequency by GABA in GAD65−/− pyramidal cells ( n =8 for 1 μM GABA, n =6 for 5 μM GABA). Error bars, s.e.m., * P <0.05, unpaired ( a , b ) and paired ( d ) t -test. Full size image Exogenous GABA increased the frequency of sIPSCs in GAD65−/− pyramidal cells (1 μM, by 1.15±0.05 Hz, n =8, P <0.001 paired t -test, and 5 μM, by 1.13±0.04 Hz, n =6, P <0.001 paired t -test, Fig. 8c,d ). Interestingly, this increase in the frequency of sIPSCs was not proportional to the increase in GAD65−/− interneuron firing, whereas 5 μM GABA increased firing frequency several times more than 1 μM ( Fig. 7e,f ). There are at least two explanations for such a discrepancy. First, using somatic recordings, we were unable to detect sIPSCs from distal dendrites, and thus the frequency change might be underestimated. Second, interneurons target both pyramidal cells and other interneurons. The output of interconnected interneurons to pyramidal cells might not exactly follow the average firing rate of individual interneurons recorded in the str. radiatum . These considerations point to the complexity of the interneuron network and the need for future studies to dissect the effect of tonic excitation on different classes of interneurons. The present data, however, are sufficient to draw the general conclusion that resting levels of ambient GABA are set to maintain the tone of synaptic GABA-mediated signalling in the hippocampal CA1 region. Changes in extracellular GABA determine the magnitude of tonic GABA A conductance, which has a biphasic effect on the excitability of hippocampal interneurons. A low-tonic GABA A conductance depolarizes the cell and results in the onset of cell firing. This depolarization also enhances voltage-dependent RMP fluctuations, which are driven by stochastic Na + channel opening [29] . It is likely that these fluctuations are involved in the increase in the cell firing rate, because they get larger following GABA A -mediated depolarization. When the tonic GABA A conductance increases, the excitatory effect of depolarization is overpowered by inhibition. Both cell firing frequency and RMP fluctuations decrease. This inhibition can be explained by the shunting effect, which increases with the tonic GABA A conductance. Consistent with the effect of shunting, evoked synaptic GABA A signalling was inhibitory in interneurons, because of the large peak conductance. This finding, however, does not rule out the possible excitatory effect of relatively small spontaneous GABA A -mediated postsynaptic currents. Nevertheless, the present finding adds one more distinction to the functional role of tonic and phasic GABA-mediated signalling in the brain [1] , [2] , [3] . A biphasic effect of tonic GABA A conductance on neuronal firing has important implications for computation within a neuronal network. The classic view holds that neurons generate a variable output in response to the integration of synaptic inputs. Here we show that hippocampal interneurons can generate a variable output in response to changes in extrasynaptic GABA, regardless of excitatory synaptic drive. Because these neurons are part of the local circuit, extrasynaptic input can be considered as one of the inputs into the local neuronal network that determines the network operation and output. An increase in ambient GABA has been reported for particular types of behaviour (for example, exploration [11] ) or in pathological conditions [10] , [12] . We used bath application of GABA to mimic such an increase. Exogenous GABA, however, also induced a dose-dependent tonic current with a magnitude of two orders larger than the time-averaged current produced by the change in sIPSCs in CA1 pyramidal neurons. Because these cells are reported to have hyperpolarizing E GABA (ref. 17 ), the tonic GABA A current may be their main source of inhibition. This raises the question of whether a biphasic change in sIPSC frequency is of any importance for the excitability of pyramidal neurons. In fact, bath application of GABA may not faithfully reproduce the changes in ambient GABA concentrations under physiological conditions. A recent report using an innovative GABA imaging technique demonstrated layer-specific changes in ambient GABA resulting from increased neuronal activity [43] . Moreover, the functional roles of tonic and phasic GABA A signalling are largely different [2] , [30] . For example, tonic GABA A conductance determines the membrane time constant and characteristic length constant [30] , and modulates neuronal offset in CA1 pyramidal neurons [44] . GABA A -mediated IPSCs interact in a time-dependent manner with glutamatergic EPSCs, which has a specific impact on neuronal computation (for example, integration time window of neuronal inputs [45] ), and are involved in network synchronization and oscillatory behaviour [46] . Thus, the actual effect of physiological changes in ambient GABA concentration on the hippocampal network function requires further investigation. In summary, we suggest that the described phenomenon has a role in different types of excitable cells. The amount of conductance acts to switch between excitation and inhibition when certain conditions are met: the current has low depolarizing reversal potential and the produced depolarization is amplified by other voltage-dependent conductances. Here we demonstrated these conditions in hippocampal interneurons, but they can be potentially observed in the other neurons with depolarizing E GABA (refs 9 , 22 , 23 , 24 , 25 ). It is also likely that E GABA determines the excitation peak conductance and the inhibitory threshold conductance. Thus, the biphasic action of tonic GABA A conductance should be considered in the broader context of the determinants of E GABA . First, the expression of the main Cl − transporters (NKCC1 and KCC2) is developmentally regulated, which differs in various cell types. For example, in hippocampal pyramidal neurons, the ratio of KCC2/NKCC1 increases during development, making GABA hyperpolarizing [14] . In contrast, this ratio is fixed in hippocampal interneurons and GABA continues to have depolarizing effects throughout development [19] . Second, activity-dependent regulation of Cl − transporters contributes to E GABA in different cells. A recent report demonstrated that NMDA receptor activity downregulates KCC2, resulting in a depolarizing GABA A -mediated current in rat dissociated neurons [47] . Additionally, the described phenomenon can have a role at subcellular level. We did not systematically investigate the effect of low GABA concentrations at different sites within interneurons. A previous report, however, demonstrated that depolarizing GABA can produce inhibition in the soma and excitation in dendrites of cortical pyramidal cells [48] . This can be explained that shunting inhibition of the axon initial segment is larger for soma than for more remote dendritic sites. That is, the inhibitory threshold conductance increases with distance from the axon initial segment. This observation prompts further investigation of tonic GABA A conductances at the subcellular level. Electrophysiology in hippocampal slices All experimental procedures were performed in accordance with the guidelines of the Animal Experiment Committee of the RIKEN Brain Science Institute. Hippocampal slices (350–380 μm) were obtained from 4- to 6-week-old male WT or GAD65−/− littermates [49] . Heterozygous knockout mice with a C57BL/6J genetic background were interbred to produce WT and GAD65−/− mice in a specific pathogen-free facility. Mice were housed at 24 °C with a 12/12-h light/dark cycle and ad libitum access to food and water. Genomic PCR was used to differentiate the mice. Hippocampal slices were maintained at room temperature in a submerged chamber with solution containing (in mM): 119 NaCl, 2.5 KCl, 1.3 MgSO 4 , 1 CaCl 2 , 26.2 NaHCO 3 , 1 NaH 2 PO 4 , and 11 glucose, and saturated with 95% CO 2 /5% O 2 . After 1 h of incubation, slices were transferred to the recording chamber and superfused at 34 °C with the solution described above, but containing 2.5 mM CaCl 2 . Except for the experiment shown in Supplementary Figure S1 , AMPA/kainate, NMDA, and GABA B receptors were blocked with 25 μM NBQX, 50 μM APV, and 5 μM CGP 52432 (Tocris Cookson), respectively. CA1 pyramidal cells and str. radiatum interneurons were visually identified with an infrared differential interference contrast microscope (Olympus BX51WI). The data were acquired with a Multiclamp700B (Axon Instruments), filtered at 2 kHz, and digitized at 5 kHz using a NI PCI-6221 data acquisition card (National Instruments). The data were analysed without further re-sampling. Sample traces were also taken at the same rate, except for the long traces (>30 s), which were re-sampled at 10 Hz. Whole-cell, gramicidin-perforated patch, and cell-attached recordings were performed in separate cells. Whole-cell experiments Whole-cell pipettes used in voltage-clamp recordings contained (in mM): 130 CsCl, 8 NaCl, 10 Cs-HEPES, 2 EGTA, 0.2 MgCl 2 , 2 MgATP, 0.3 Na 3 GTP, and 5 QX314Br (pH 7.2, osmolarity 295 mOsm, liquid junction potential 4.1 mV). In the experiments for Figure 7a , KCl was used instead of CsCl (liquid junction potential 3.4 mV). Whole-cell current-clamp recordings were performed with pipettes containing (in mM): 132.3 K-gluconate, 7.7 KCl, 4 NaCl, 0.5 CaCl 2 , 10 HEPES, 5 EGTA, 2 MgATP, and 0.5 Na 3 GTP. Series resistance ( R s ), input resistance ( R i ), and membrane capacitance ( c m ) were monitored throughout the recordings. These parameters were obtained from the current in response to hyperpolarizing voltage steps ( V step =−5 mV). where, I peak is the peak amplitude of the current transient immediately after the step is applied, is the decay time constant of the current, and I ss is the steady-state current [50] . The R s was not compensated and data were discarded if R s changed by more than 20% during the recording. There was no significant difference in c m between GAD65−/− (70.9±7.9 pF, n =9) and WT (69.4±6.9 pF, n =11) interneurons ( P =0.445). Tonic GABA A current ( I tonic ) was calculated as the difference between the baseline I hold and the I hold in the presence of a GABA A receptor antagonist. The change in the tonic GABA A current (Δ I tonic ) was calculated as the difference between the baseline I hold and the I hold in the presence of exogenous GABA. I tonic density was obtained by dividing I tonic by the surface area of the neuron. The surface area was obtained by dividing c m by the membrane capacitance constant (0.9 μF cm -2 ) [50] . Tonic GABA A conductance was calculated as the difference between the baseline conductance (1/ R i ) and the conductance in the presence of a GABA A receptor antagonist ( g GABA ) or exogenous GABA (Δ g GABA ). Synaptic GABA A conductance in response to electric stimulation (PSG, Fig. 3a ) was calculated according to where PSC—postsynaptic current in the presence of ionotropic glutamate and GABA B receptor antagonists; V hold =70 mV—holding current; E GABA =−0.7 mV was calculated by where P Cl =1 and p HCO 3 = 0.2−relative permeabilities for Cl − and HCO 3 − , respectively [51] . mISPCs were recorded in the presence of 1 μM tetrodotoxin. sIPSCs and mIPSCs were completely blocked by 100 μM picrotoxin. Frequency, mean amplitude, and decay time constant of sIPSCs and mIPSCs were analysed off-line with the MiniAnalysis (Synaptosoft) and Clampfit (MDS Analytical Technologies). aIPSC frequency was calculated as the difference between the sIPSC and mIPSC frequencies. Time-averaged current mediated by sIPSCs ( I spont ) was calculated as the mean charge transfer of sIPSCs multiplied by their frequency [6] . Gramicidin-perforated patch experiments The pipette tips were filled with the solution containing (in mM) 145 KCl, 10 HEPES, 5 ATP-Mg, 0.2 GTP-Na, 2 QX314, and 2 EGTA to prevent leakage of the antibiotic while approaching the cell. The pipettes were back-filled with the same solution that also contained 20 μg ml −1 gramicidin-D (Sigma). Fresh gramicidin solution was made every 2 h. After the pipette tip contacted the cell membrane, the R s was monitored. Recordings were started when the R s stabilized at 30–45 MΩ (usually within 15–20 min). All measurements were corrected for a liquid junction potential and voltage drop across the R s (ref. 52 ). RMP was measured in current clamp mode ( I hold was 0 pA). Mean RMP and its standard deviation were obtained under control conditions and in the presence of GABA. The depolarizing effect of GABA was calculated as difference between mean RMPs. In some experiments, the cells were voltage-clamped at −65 mV. Membrane I–V characteristics were then obtained with 2,000-ms voltage steps delivered from −90 to −70 mV with 10 mV intervals, and from −55 to −20 mV with 5-mV intervals. I–V characteristics for GABA A tonic current were obtained as the difference between membrane I–V characteristics in 5 μM GABA and in 100 μM picrotoxin, added sequentially. Cell-attached experiments Pipettes were filled with superfusion solution and loosely attached to the cell membrane to measure interneuron firing without perturbing intracellular ionic concentrations. Recordings were performed in the voltage-clamp mode from the interneurons in which action currents were detectable (approximately 50% of cells) [21] , [27] . The command potential was set to the potential at which the holding current was 0 pA to avoid direct cell stimulation by the electrode [53] . The evoked GABA A -mediated PSGs were triggered by 200-μs current pulses at 50 μA delivered by a tungsten monopolar electrode placed in the str. radiatum . GABA A activation was also produced with a 100-μM GABA puff (100 ms, 50 psi). Preceding ( t ps ) and succeeding ( t ss ) spike intervals were calculated from the beginning of the synaptic stimulation or GABA puff. Computational model The cylindrical neuron (length 20 μm; diameter 10 μm; total surface 628 μm 2 ) was created with the Neuron 7 simulator. The cell excitability was described according to Hodgkin–Huxley's model with corresponding Na + (Na v ) and K + (K v ) channels (single-channel conductance: γ Na =20 pS and γ K =15 pS; channel density: 50 and 0.667 μm −2 , giving a total number of channels of N Na =31,400 and N K =419). Additionally, A-type K + channels ( K A ) were introduced (single-channel conductance γ KA =10 pS; channel density: 8 μm −2 giving total number of channels: N KA =5,024) [34] . The transition of the channels between different conformational states was described as a Markov process, whereas the rate constants varied with the voltage [54] , [55] . The membrane also included the linear deterministic tonic GABA A conductance ( g GABA ), which was varied from 0 to 0.2 mS cm -2 with 0.001 mS cm -2 steps. On the basis of this set of conductances, we used the following equation: where C m —membrane capacitance (1 μF cm -2 ), I inj —injected current (0 pA for baseline conditions), E Na —Na + equilibrium potential (50 mV), and E K —K + equilibrium potential (−77 mV). The reversal potential for GABA A current ( E GABA =−55 mV) was set 10.2 mV above the mean RMP without GABA A conductance (65.2 mV) to match experimental data. g Na , g K , and g KA —Na V , K V , and K A conductances, respectively, were controlled by continuous variables that range between 0 and 1 ( m , h , n , k , l ). where [ m 3 h 1 ], [ n 4 ], and [ l 1 k 1 ] are the probabilities of the Na V , K V , and K A channels to be in the open state according to their respective kinetic schemes [54] , [55] . The variables m , h , n , k , l obeyed first-order differential equations with voltage dependent rate constants ( α m , β m , α h , β h , α n , β n , α k , β k , α l ). The effect of g GABA on fluctuations of RMP (RMP standard deviation) was studied when the density of Na + channels was reduced from 50 to 25 μm −2 to prevent action potential generation. The effect of membrane depolarization on the cell firing and the RMP fluctuations was studied with the current injections ( I inj ) from 0 to 1 nA and g GABA =0 nS. All simulations were run for 1,000 ms, and the data were collected from the interval between 500 ms and 1,000 ms when the model reached a quasi-steady state. All the model data are means from 10 independent simulations. To avoid the correlation between data, each computation was performed with a different seed obtained from the random number generator. Statistical analysis Data are presented as means±s.e.m. Error bars on the graphs represent s.e.m. Statistical comparisons were made using unpaired Student's t -test unless a paired t -test is stated. A P -value of less than 0.05 was considered statistically significant. A.S. and I.S. designed the study and planned the experiments; A.S., I.S., and L.S. analysed the data and prepared the manuscript; I.S. performed all the experiments; L.S. performed the modelling. How to cite this article: Song, I. et al . Tonic excitation or inhibition is set by GABA A conductance in hippocampal interneurons. Nat. Commun. 2:376 doi: 10.1038/ncomms1377 (2011).